High current superconductivity in FeSe0.5Te0.5-coated conductors at 30 tesla Although high-temperature superconductor cuprates have been discovered for more than 25 years, superconductors for high-field application are still based on low-temperature superconductors, such as Nb 3 Sn. The high anisotropies, brittle textures and high manufacturing costs limit the applicability of the cuprates. Here we demonstrate that the iron superconductors, without most of the drawbacks of the cuprates, have a superior high-field performance over low-temperature superconductors at 4.2 K. With a CeO 2 buffer, critical current densities >10 6 A cm −2 were observed in iron-chalcogenide FeSe 0.5 Te 0.5 films grown on single-crystalline and coated conductor substrates. These films are capable of carrying critical current densities exceeding 10 5 A cm −2 under 30 tesla magnetic fields, which are much higher than those of low-temperature superconductors. High critical current densities, low magnetic field anisotropies and relatively strong grain coupling make iron-chalcogenide-coated conductors particularly attractive for high-field applications at liquid helium temperatures. Iron-based superconductors are semi-metallic materials with transition temperatures, T c , up to 55 K. The combination of extremely high upper critical fields, H c2 (0) (estimated to be on the order of 100 T), moderate H c2 ab /H c2 c anisotropies (on the order of 1–8) and high irreversibility fields, H irr , makes this class of superconductors particularly appealing for high-field applications [1] , [2] , [3] , [4] , [5] , [6] , [7] , [8] , where the critical current density, J c , is a major limiting factor. Although the high- T c cuprates currently hold the records of J c value among all superconductors, there are quite a few obstacles for their practical application. The extremely high anisotropies up to thousands have made it very difficult to obtain superconducting tapes or wires with their best J c . The rapid decrease of J c upon the grain boundary misorientation also made their fabrication much more difficult and complicated. Their brittle textures as well as the high production and raw material costs also hold back their application. Currently, superconductors for high-field application are still based on Nb 3 Sn, a low T c superconductor that allows fields in excess of 20 T to be achieved at 4.2 K. We argue that iron superconductors may be a more competitive candidate to replace these low T c superconductors for high-field application at liquid helium temperatures. To achieve this goal, a key task is to find a technique to increase the J c of iron-superconductor films (or wires) made on practical metal substrates (or inside metal sheath). One of these techniques is to make a proper buffer layer between the superconductor and the substrate. A suitable buffer layer can often prevent undesirable reactions between the superconductor and the substrate, or enhance the superconducting properties of the films and wires. For iron-pnictide films, Tarantini et al . [9] recently reported that single-crystalline (La, Sr)(Al, Ta)O 3 substrates with 100 unit cells of epitaxial SrTiO 3 (STO) resulted in higher T c and J c for Co-doped BaFe 2 As 2 films. Higher T c and sharper out-of-plane and in-plane textures of the Fe/BaFe 2 As 2 bilayers were also realized with 20-nm thick epitaxial Fe buffer layers [10] . A self-field J c >1 MA cm −2 at 4.2 K has been reported in both Co-doped BaFe 2 As 2 and SmFeAs(O, F) systems [1] , [2] , as well as in Co-doped BaFe 2 As 2 thin films on coated conductor substrates [4] . However, the results of high-field performance up close to their H irr at 4.2 K are still missing. Here we show that epitaxially grown iron-chalcogenide thin films with a CeO 2 buffer layer have a superior high-field performance up to 30 T with J c >1 MA cm −2 in self-field. Chalcogenides are an interesting sub-class of iron-based superconductors. Even though the T c of chalcogenides are typically <20 K, it was found that the T c of FeSe can reach 37 K under a pressure of ~7 GPa (ref. 11 ). Recently, it was reported that a single-unit cell film of FeSe on a STO substrate may be superconducting >77 K (ref. 12 ). They also have the simplest structures among the iron-based superconductors and exhibit lower anisotropies ~2, compared with the pnictides, with comparable H c2 (0) approaching 50 T (refs 13 , 14 , 15 ). We have previously reported on the successful growth of FeSe 0.5 Te 0.5 (FST) thin films on textured metal templates with biaxially aligned MgO layers, made via ion-beam-assisted deposition (IBAD) [3] . These films carry J c >10 4 A cm −2 under magnetic fields as high as 25 T at about 4 K. However, MgO has a cubic lattice constant of ~4.11 Å, which is fairly larger than the in-plane lattice constant of FST, which is around 3.81 Å. CeO 2 , a commonly used buffer layer for high-temperature superconductor (HTS) cuprates, has a much closer lattice constant (cubic, ) with FST. In this article, we show that CeO 2 buffer can significantly improve the T c and J c of FST films both on single-crystalline substrates and coated conductors, such as the rolling-assisted biaxially textured substrate (RABiTS), which have a biaxially textured CeO 2 layer at the top [16] . These films have a self-field J c as high as 1 MA cm −2 and maintain a nearly isotropic J c on the order of 1 × 10 5 A cm −2 up to 30 T at 4.2 K. 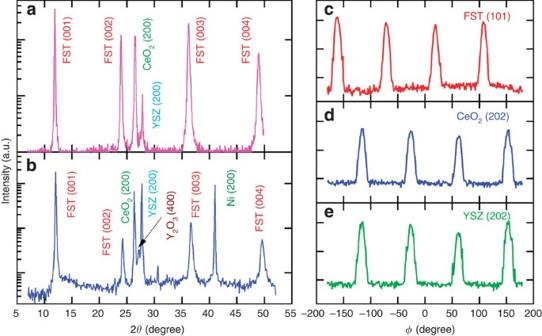Figure 1: Structure analysis of FST films by XRD. θ-2θscan of FST films grown on (a) a YSZ single-crystalline substrate with CeO2buffer layer and (b) a RABiTS substrate.φscan of (c) (101) peak from the FST film, (d) (202) peak from the CeO2buffer layer and (e) (202) peak from YSZ buffer layer in a FST film grown on a RABiTS subtrate. Both the film and buffer layers are well aligned in-plane and out-of-plane. The lattice of the FST film is rotated by 45° in theabplane compared with the lattice of CeO2/YSZ buffer layers. Structure of FST films on CeO 2 -buffered substrates Figure 1a shows a θ -2 θ X-ray diffraction (XRD) scan of a typical FST film grown on a (100) Yttria-stabilized zirconia (YSZ) substrate with a buffer layer of CeO 2 . Figure 1b shows the same scan for a film grown on a RABiTS substrate. For both films, only the (00 l ) peaks from the FST film, CeO 2 buffer and substrates are present, indicating that the out-of-plane alignments are good. The CeO 2 , YSZ and Y 2 O 3 layers, with the NiW base layer, in the RABiTS substrate are clearly seen in the XRD scan. Figure 1c–e shows the φ scan of the (101) peak from the thin film and the (202) peak from the CeO 2 and YSZ buffer layers in the RABiTS substrate. All of them have four peaks with 90° intervals consistent with four-fold symmetry. Peaks from the thin film and the CeO 2 /YSZ buffer layers are separated by 45°, indicating that the lattice of the film is rotated by 45° in the ab plane compared with the lattice of CeO 2 /YSZ buffer layers and is now aligned cube-on-cube with the NiW substrate. The c -axis lattice constant is about 5.90–5.94 Å for both types of films, which is shorter than that of the bulk sample (6.02 Å). This is consistent with our previous results from films grown on other substrates [3] , [17] . Figure 1: Structure analysis of FST films by XRD. θ -2 θ scan of FST films grown on ( a ) a YSZ single-crystalline substrate with CeO 2 buffer layer and ( b ) a RABiTS substrate. φ scan of ( c ) (101) peak from the FST film, ( d ) (202) peak from the CeO 2 buffer layer and ( e ) (202) peak from YSZ buffer layer in a FST film grown on a RABiTS subtrate. Both the film and buffer layers are well aligned in-plane and out-of-plane. The lattice of the FST film is rotated by 45° in the ab plane compared with the lattice of CeO 2 /YSZ buffer layers. 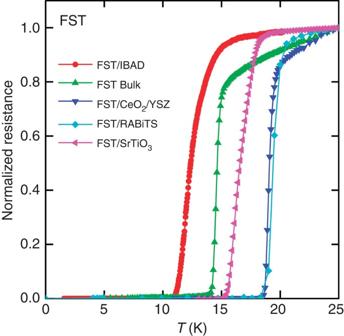Figure 2: Resistive superconducting transition of various FST films and the bulk material. Tcof FST films (except for that grown on the IBAD substrate) are 2–5 K higher than that of bulk. Films with CeO2buffer layers have the highestTcwith an onsetTc>20 K and zero resistanceTc>18 K. Full size image T c comparison of various FST films and the bulk material Figure 2 shows the resistive superconducting transitions of various FST thin films and the bulk material. It is clearly seen that FST films (except for that grown on IBAD substrates) have T c 2–5 K higher than that of bulk. The highest T c is achieved with a CeO 2 buffer layer, which has an onset T c >20 K and zero resistance T c >18 K. The transition width (10–90% normal resistance level) is under 1 K. The most striking finding is that the film grown on RABiTS has a higher T c than the film grown on single-crystalline substrate without a CeO 2 buffer layer, although the latter actually has a smaller in-plane texture. The full-width half maximum of the (101) peak from the φ scan (Δ φ 101 ) is about 6°, which is smaller than the CeO 2 texture in the RABiTS substrate (Δ φ 202 ~7°). This behaviour was also observed in Ba(Fe 1− x Co x ) 2 As 2 films by Katase et al . [4] However, Δ φ 101 for films on single-crystalline substrates without a CeO 2 buffer are just ~2°. Even films on IBAD substrates have better textures (Δ φ 101 ~5°) (ref. 3 ). These results suggest that the CeO 2 buffer has a much more profound effect on the superconducting properties of FST thin films than the sharpness of the texture in the films themselves. Films on IBAD substrates have the lowest T c (~11 K) as shown in Fig. 2 . This is probably due to its largest lattice mismatch to the FST [3] . Figure 2: Resistive superconducting transition of various FST films and the bulk material. T c of FST films (except for that grown on the IBAD substrate) are 2–5 K higher than that of bulk. 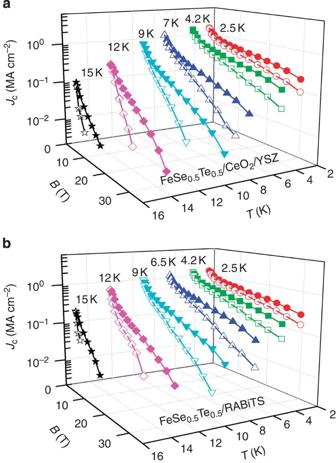Figure 3: Critical current densities (Jc) of FST films. Jcof FST films on (a) a YSZ substrate with a CeO2buffer layer and (b) a RABiTS substrate at various temperatures with magnetic field parallel (solid symbols) and perpendicular (open symbols) to theabplane (tape surface). The self-fieldJcof both films are above 1 MA cm−2at 4.2 K. Under 30 T of magnetic fields, both films still carryJcaround 1 × 105A cm−2. Films with CeO 2 buffer layers have the highest T c with an onset T c >20 K and zero resistance T c >18 K. Full size image J c of FST films Figure 3 shows the magnetic field dependence of the J c of the FST films grown on both CeO 2 -buffered single-crystalline YSZ and RABiTS substrates at various temperatures. The J c of films grown on both substrates are shown to be >1 MA cm −2 in self-field at 4.2 K, and remain on the order of 1 × 10 5 A cm −2 up to 31 T—the maximum field we could apply. Notably, the decrease of J c does not accelerate much at high fields at liquid helium temperatures, which is important for high-field magnet applications. Surprisingly, the J c of the RABiTS film under higher magnetic fields or at higher temperatures is somehow higher than those of films on single-crystalline substrates, although the film grown on the RABiTS substrate has a macroscopic 6° in-plane misalignment of epitaxial grains, which is much higher than that of the film grown on single-crystalline substrates. It has been well known that a key factor limiting the applications of HTS wires is the high-angle grain boundaries that cause the rapid decrease of J c . Our X-ray texture analysis indicates an average 7° grain boundary misalignment in the RABiTS substrates we used. It is interesting to note that very high J c of >3 MA cm −2 (77 K, self-field) with well-linked behaviour is routinely obtained for YBa 2 Cu 3 O 7 (YBCO) films on these substrates. This seems to be the case in the FST films. Our observation is markedly different from an earlier report on grain boundaries of Ba(Fe 1− x Co x ) 2 As 2 films, which shows that grain boundaries could significantly reduce the J c even at low angles [18] . A recent report on films of iron-based superconductors by Katase et al . [19] has shown that the critical angle for the rapid J c decrease is about 9°. This is consistent with our studies, although their films are pnictides, whereas our films are chalcogenides. Figure 3: Critical current densities ( J c ) of FST films. J c of FST films on ( a ) a YSZ substrate with a CeO 2 buffer layer and ( b ) a RABiTS substrate at various temperatures with magnetic field parallel (solid symbols) and perpendicular (open symbols) to the ab plane (tape surface). The self-field J c of both films are above 1 MA cm −2 at 4.2 K. Under 30 T of magnetic fields, both films still carry J c around 1 × 10 5 A cm −2 . Full size image In Fig. 4a , we show the field dependence of the volume pinning force F p for a FST film grown on a RABiTS substrate with the literature data of the second-generation YBCO wire [20] , [21] , thermomechanically processed Nb47Ti alloy [22] , [23] and small-grain Nb 3 Sn wire [24] , [25] . Clearly, the FST film exhibits superior high-field performance (above ~7 T) over those of other low-temperature superconductors. YBCO and other HTSs currently have higher J c than the ones typical of iron chalcogenides, but their applications are impeded by high production costs, higher anisotropies, and the rapid decrease of J c upon grain boundary misorientation. We noted that the cost of the coated conductors mainly depends on the cost of the processing methodologies, not the raw materials. This cost is mostly related to the growth of the thick multiple textured oxide buffer layers, partially to prevent metal template from oxidation, as well as the sophisticated procedures necessary for growing YBCO films near 800 °C and the oxygen annealing afterwards. For the new iron-based coated conductors, the processing temperature is much lower (~400°C) (ref. 17 ). At this moderate temperature, we expect very limited oxidation of the metal templates, hence thinner and less-complicated buffer structures are likely to produce the same result. Furthermore, oxygen annealing is no longer required. As such, we expect the manufacturing cost of iron-based coated conductors will be reduced, which may make them more attractive on the cost-performance basis. 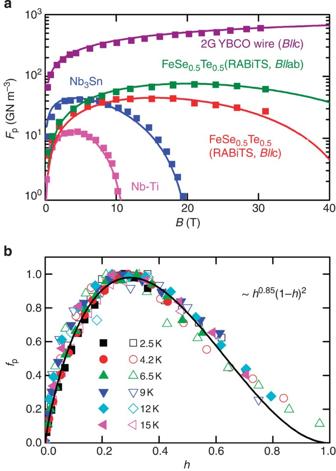Figure 4: Pinning force analysis for a FST film grown on RABiTS. (a)Fpat 4.2 K of a FST film grown on a RABiTS substrate, compared with the literature data of YBCO 2 G wire20,21, TCP Nb47Ti22,23and Nb3Sn24,25. Solid lines are Kramer’s scaling approximations. (b)Kramer’s scaling of pinning force densityfpversus reduced fieldhfor a FST film grown on a RABiTS substrate at various temperatures with field perpendicular (solid symbols) and parallel (open symbols) toc-axis. Figure 4: Pinning force analysis for a FST film grown on RABiTS. ( a ) F p at 4.2 K of a FST film grown on a RABiTS substrate, compared with the literature data of YBCO 2 G wire [20] , [21] , TCP Nb47Ti [22] , [23] and Nb 3 Sn [24] , [25] . Solid lines are Kramer’s scaling approximations. ( b) Kramer’s scaling of pinning force density f p versus reduced field h for a FST film grown on a RABiTS substrate at various temperatures with field perpendicular (solid symbols) and parallel (open symbols) to c -axis. Full size image In Fig. 4b , we show the Kramer’s scaling law approximation (solid line), f p ~ h p (1− h ) q , for a FST film grown on a RABiTS substrate at various temperatures with the field applied both parallel and perpendicular to the tape surface, where f p = F p / F p max is the normalized pinning force density and h = H / H c2 is the reduced field. The data for all temperatures and both directions fall approximately on a single line. This appears to suggest that the pinning mechanism is independent of the temperature and field direction. q is found to be equal to 2, which is expected considering that the (1− h ) [2] term describes the reduction of the superconducting order parameter at high fields [26] . p is found to be ~0.85 ( h 0.85 ), close to 1. This low-field term indicates that a point-defect core pinning mechanism is at play [26] , which is consistent with our previous results of FST films grown on IBAD substrates [3] . In the core pinning regime, F p is a product of the individual F p times the pinning centre density. This means that the J c of FST may still be enhanced by adding more defects to act as pinning centres. It is not clear what types of defects are responsible for the high J c values we observed so far, in particular, what is the role of the CeO 2 buffer layer. We attempted to answer these questions by examining the structure properties of our FST films. Our preliminary high-resolution transmission electron microscope study revealed that there might be some intergrowth at the interface between the FST films and the CeO 2 buffer layers. We noted that certain types of intergrowth defects can be effective flux pinning centres in cuprates [27] . Perhaps, they also contribute to the enhanced pinning observed in the FST films on the CeO 2 buffer layers, and result in significantly improved J c . To understand the flux pinning mechanism, a detailed study of the structure–properties relationship is needed. This is our ongoing effort, and findings will be reported elsewhere. In conclusion, robust c -axis oriented superconducting FST tapes on CeO 2 -buffered single-crystalline and RABiTS coated conductor substrates have been made by pulsed-laser deposition. These tapes have a self-field J c on the order of 1 MA cm −2 and carry a nearly isotropic J c ~10 5 A cm −2 under 30 T at 4.2 K. The CeO 2 buffer layer dramatically improves the superconducting performance of the FST films. It was also found that the low-angle (up to 7°) substrate grain boundary does not depress the J c of the coated conductor films. These properties show that FST has a very promising future for high-field applications at liquid helium temperatures. We used pulsed-laser deposition to grow the FST films and CeO 2 buffer layers [17] . Films were deposited on both single-crystalline substrates, such as LaAlO 3 , STO and YSZ, and RABiTS. RABiTS substrates were originally developed and are presently being used extensively in the production of high- T c cuprate films. They are comprised of a Ni–W alloy with a series of buffer materials, such as Y 2 O 3 , YSZ and CeO 2, on top. The topmost is a biaxially textured CeO 2 layer with an in-plane texture of about 7° [16] . Structural characterizations of the various films were performed by XRD at beamline X18A at the National Synchrotron Light Source at Brookhaven National Laboratory. The beam energy is 10 keV. The resistivities and the J c were measured utilizing a standard four-probe method. Experiments at magnetic fields as high as 31 T were conducted at the National High Magnetic Field Laboratory in Tallahassee, Florida. How to cite this article : Si, W. et al . High current superconductivity in FeSe 0.5 Te 0.5 -coated conductors at 30 tesla. Nat. Commun. 4:1347 doi: 10.1038/ncomms2337 (2013).